PAR-CLIP analysis uncovers AUF1 impact on target RNA fate and genome integrity Post-transcriptional gene regulation is robustly regulated by RNA-binding proteins (RBPs). Here we describe the collection of RNAs regulated by AUF1 (AU-binding factor 1), an RBP linked to cancer, inflammation and aging. Photoactivatable ribonucleoside-enhanced crosslinking and immunoprecipitation (PAR-CLIP) analysis reveals that AUF1 primarily recognizes U-/GU-rich sequences in mRNAs and noncoding RNAs and influences target transcript fate in three main directions. First, AUF1 lowers the steady-state levels of numerous target RNAs, including long noncoding RNA NEAT1 , in turn affecting the organization of nuclear paraspeckles. Second, AUF1 does not change the abundance of many target RNAs, but ribosome profiling reveals that AUF1 promotes the translation of numerous mRNAs in this group. Third, AUF1 unexpectedly enhances the steady-state levels of several target mRNAs encoding DNA-maintenance proteins. Through its actions on target RNAs, AUF1 preserves genomic integrity, in agreement with the AUF1-elicited prevention of premature cellular senescence. In mammalian systems, post-transcriptional mechanisms govern gene expression programs across cell types, developmental stages and metabolic conditions. By controlling pre-mRNA splicing and maturation, as well as mRNA transport, storage, editing, turnover and translation, post-transcriptional processes influence the type, abundance and location of expressed proteins. These steps are governed by two main types of RNA-interacting factors acting in concert: noncoding (nc)RNAs and RNA-binding proteins (RBPs) [1] , [2] . The vast class of ncRNAs includes small RNAs (notably microRNAs), which generally function as repressors of mRNA stability and/or translation [3] , and long (l)ncRNAs, which also modulate target mRNA turnover and translation [4] . The other large family of regulatory factors, RBPs, affects all post-transcriptional levels of gene expression. Each individual RBP frequently influences more than one area of gene regulation, for example, RBPs HuR and HuD control the splicing, stability and translation of different target mRNAs, NF90 controls primarily bound mRNA stability and translation and nucleolin participates in transport, maturation, storage, turnover and translation of target transcripts [5] , [6] , [7] . Through these actions, RBPs and ncRNAs influence a wide range of cellular processes (for example, cell proliferation, apoptosis, autophagy, motility and the stress and immune responses) that impact on a variety of physiologic and disease processes [7] , [8] , [9] , [10] . The RBP AUF1 (AU-rich element-binding factor 1), also known as hnRNP D (heterogeneous nuclear ribonucleoprotein D), comprises four different isoforms (p37, p40, p42 and p45) that arise through alternative splicing; all of them have two RNA-recognition motifs through which they bind RNA as AUF1 monomers or oligomers [11] , [12] . AUF1 member proteins are generally considered to promote the decay of many target mRNAs, which have been identified over the years. They include mRNAs that encode cell cycle-regulatory proteins (cyclin D1, p21, p27, p16 and pRB), oncoproteins (FOS, JUND and MYC), apoptosis-related proteins (BCL2 and BAX) and inflammatory factors (such as interleukin (IL) -1β, -6, -8, granulocyte–macrophage colony-stimulating factor and tumour necrosis factor alpha (TNFα)). At least in part through these interactions, AUF1 was implicated in cellular processes such as proliferation, senescence and the response to immune and stress agents [11] , [12] . AUF1 has also been associated with decreased carcinogenesis (for example, by suppressing the expression of BCL2 or cyclin D1), however, AUF1 levels are elevated in many malignancies, including sarcomas, lymphomas and carcinomas, and has been proposed to contribute to cancer pathogenesis [13] . In other disease states, AUF1-knockout mice develop atopic dermatitis and experience severe endotoxic shock following exposure to lipopolysaccharide; these effects were attributed to the presence of constitutively elevated TNFα and IL-1β, since the mice could not degrade the mRNAs encoding these cytokines [14] , [15] . Moreover, AUF1 knockout displayed a phenotype of accelerated aging linked to enhanced telomere erosion, increased levels of inflammatory cytokines and the accumulation of senescent cells [16] . Considering the phenotypes elicited by altering AUF1 status, there is escalating interest in characterizing the molecular actions of AUF1 in full. Besides its well-established decay-promoting function, AUF1 also stabilized certain target mRNAs, including the parathyroid hormone ( PTH ), the von Hippel–Lindau ( VHL ) and the methionine adenosyltransferase 1A ( MAT1A ) mRNAs [17] , [18] , [19] , and modulated the translation of other mRNAs [20] , [21] . Moreover, evidence is accumulating that the different AUF1 isoforms may have distinct structure, localization, target RNA preference and impact on gene expression patterns [13] . In addition to its strong affinity for AU-rich RNA sequences, AUF1 also interacts with G-rich RNAs, such as the RNAs present in telomeric sequences [22] , [23] . Thus, AUF1 is expected to bind to a heterogeneous subset of RNAs and to have a variety of effects. To investigate systematically the complex functions of AUF1, we sought to identify the entire collection of RNAs bound to each isoform, as well as the precise sites of interaction. Techniques that measured AUF1 binding to recombinant RNAs (for example, RNA electrophoretic mobility shift assay, pulldown of biotinylated RNA, in vitro crosslinking and immunoprecipitation (IP) and fluorescence anisotropy) [24] , [25] , [26] have shown that AUF1 interacts with AU-rich RNAs, but often examined only a single mRNA or small parts of the mRNA. Other methods to assess en masse binding of AUF1 to endogenous mRNAs (for example, RNP IP or RIP) followed by microarray analysis (RIP chip) [25] have also been informative, but the sites of interaction on precursor mRNAs as well as with ncRNAs could not be identified and rearrangement of AUF1-RNA complexes after cell lysis could not be fully excluded. Therefore, we carried out photoactivatable ribonucleotide-enhanced crosslinking and IP analysis (PAR-CLIP) to map the interactions of AUF1 with all target RNAs and to obtain highly precise sequence resolution of these interactions [27] . In PAR-CLIP, cells are cultured with a modified nucleotide (for example, 4-thiouridine) that is incorporated into newly synthesized RNAs, exposure to ultraviolet light crosslinks the RNPs and the presence of the modified ribonucleotides provides an internal control for the binding events [27] . Using PAR-CLIP analysis, we found that AUF1 associated most often with the 3′-untranslated regions (UTRs) of mRNAs and introns, and that the sites of interaction were highly U- and GU-rich (not AU rich, as anticipated). In addition, we integrated AUF1 PAR-CLIP with several high-throughput analyses to gain insight into the impact of AUF1 on target RNAs: (1) parallel analysis with whole-cell RNA sequencing (RNA-Seq) revealed the influence of AUF1 on the steady-state levels of mRNAs and ncRNAs, (2) comparison with HuR PAR-CLIP identified systematic transcripts co-regulated by the two RBPs and (3) ribosome profiling analysis informed on the consequences of AUF1 binding on target mRNA translation. From these data, a role emerged for AUF1 in the maintenance of DNA integrity, in agreement with the enhanced aging and senescence triggered by impairment of AUF1 function. AUF1 binds distinct coding and ncRNA sequences We utilized the method PAR-CLIP [27] to identify RNA targets of the RBP AUF1, which comprises four isoforms p37, p40, p42 and p45. PAR-CLIP analysis was carried out in human embryonic kidney (HEK293) cells expressing each of the epitope-tagged AUF1 isoforms at levels two- to threefold higher than endogenous AUF1 ( Fig. 1a,b ); HEK293 cells were chosen because the PAR-CLIP methodology has been optimized in this cell type [27] . RNA fragments bound to each AUF1 isoform were converted to complementary DNA after adaptor ligations, and subsequent high-throughput sequencing was performed with an Illumina platform. The resulting sequence reads were mapped to the human genome (HG19), and grouped them by overlaps using the PARalyzer software [28] , [29] . As RBPs HuR and AUF1 shared affinity for several target mRNAs [30] , [31] , we also reran PARalyzer for the HuR PAR-CLIP data set [29] . Groups of overlapping PAR-CLIP sequence reads were considered binding sites if they (1) passed thresholds of ≥0.25 for T-to-C conversion frequency, (2) contained more than five reads with T-to-C conversion (one mismatch maximum allowed per read) and (3) showed at least two independent T-to-C conversions ( Supplementary Fig. 1a,b ). We obtained 86,833 binding sites of 30 nt average length in sum for all four AUF1 isoforms. 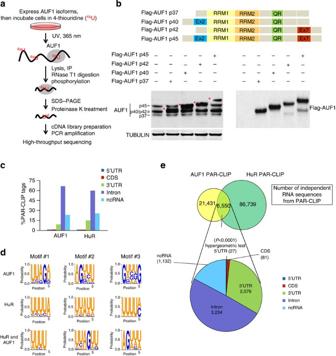Figure 1: Identification of AUF1 target RNA sequences using PAR-CLIP analysis. (a) Schematic of PAR-CLIP analysis. (b) Expression levels in transfected HEK293 cells (left) and domain organization (right) of each AUF1 isoform. Levels of endogenous AUF1 (p37, p40, p42 and p45 isoforms indicated) and ectopic Flag-AUF1 48 h after transfection as detected by western blot analysis of total AUF1, Flag and loading control α-TUBULIN; tagged AUF1 (marked with *) is slightly larger than endogenous AUF1 (Supplementary Fig. 7). (c) Percentage of AUF1 and HuR PAR-CLIP tags in mature mRNAs, introns and ncRNAs. (e) Schematic of shared binding sites among AUF1 and HuR PAR-CLIP libraries; the significance (P) of the overlap is indicated. (d) Representative (top three) RREs from AUF1 and HuR PAR-CLIP. For the most abundantly covered AUF1 p45 isoform, 33,587 binding sites distributed over 2,108 mRNAs ( Supplementary Table 1 ; Fig. 1a,b ). Similar to the HuR data set, for all AUF1 isoforms, 66.8% of mRNA-binding sites were found in intronic regions and the rest mainly in the 3′UTR ( Fig. 1c ; Supplementary Fig. 1c ), reflecting the predominantly nuclear localization of AUF1. Given that many of the binding sites of all four AUF1 isoforms overlapped, particularly when considering 3′UTR binding sites ( Supplementary Table 1 ; Fig. 1d ), we concluded that the lower number of detected binding sites for the p37 and p40 isoforms reflected a low saturation of the PAR-CLIP experiment rather than differential targeting of mRNAs. In this regard, p37 and p40 are the two AUF1 isoforms best associated with increased mRNA decay, and thus their target transcripts might be under-represented because they are preferentially degraded. Figure 1: Identification of AUF1 target RNA sequences using PAR-CLIP analysis. ( a ) Schematic of PAR-CLIP analysis. ( b ) Expression levels in transfected HEK293 cells (left) and domain organization (right) of each AUF1 isoform. Levels of endogenous AUF1 (p37, p40, p42 and p45 isoforms indicated) and ectopic Flag-AUF1 48 h after transfection as detected by western blot analysis of total AUF1, Flag and loading control α-TUBULIN; tagged AUF1 (marked with *) is slightly larger than endogenous AUF1 ( Supplementary Fig. 7 ). ( c ) Percentage of AUF1 and HuR PAR-CLIP tags in mature mRNAs, introns and ncRNAs. ( e ) Schematic of shared binding sites among AUF1 and HuR PAR-CLIP libraries; the significance ( P ) of the overlap is indicated. ( d ) Representative (top three) RREs from AUF1 and HuR PAR-CLIP. Full size image We applied cERMIT to define the in vivo RNA recognition element (RRE) for AUF1 (ref. 32 ). The three highest-scoring motifs did not contain the expected AU-rich sequences but instead were generally GU- or UG-rich; this nucleotide composition was observed regardless of the mRNA region where the PAR-CLIP tags were identified ( Supplementary Fig. 2 ). These RREs are distinct from HuR RREs, which bear four Us. However, HuR and AUF1 shared exactly the same RNA sequence at striking 6,550 sites (7% of HuR hits, 23% of AUF1 hits); these shared binding sites map mainly to introns and 3′UTRs and contain four or five Us ( Fig. 1d ; Supplementary Fig. 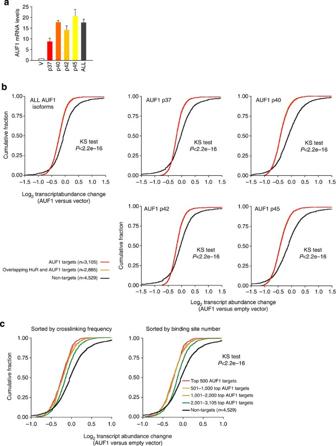Figure 2: AUF1 lowers the levels of target mRNA subsets. (a) Relative overexpression of each AUF1 isoform, as assessed by RT-qPCR analysis; data are the means+s.d. from three independent experiments. (b) Cumulative distribution analysis in abundance of AUF1 PAR-CLIP target mRNAs after AUF1 overexpression. The red lines are almost exactly superimposed on the orange lines. (c) Cumulative distribution analysis of 3,105 AUF1 target mRNAs binned by target site number or T-to-C frequency. Significance in graphs inb,cwas determined using the KS (Kolmogorov–Smirnov) test. 1e,f ; Supplementary Table 2 ; Supplementary Note ). Collectively, AUF1 and HuR share many target RNAs, suggesting a possible co-regulation of common target RNAs by these two RBPs. AUF1 reduces the levels of a subset of target mRNAs Since AUF1 shares common binding sites with HuR ( Fig. 1e ; Supplementary Fig. 1f ), an RBP that affects the stability of many target transcripts, we sought to study systematically the impact of AUF1 on target mRNA abundance on a transcriptome-wide scale. Thus, we measured mRNA abundance using RNA-Seq analysis in HEK293 cells after overexpression of all four isoforms of AUF1 using plasmid vectors and compared it with cells transfected with a control plasmid. 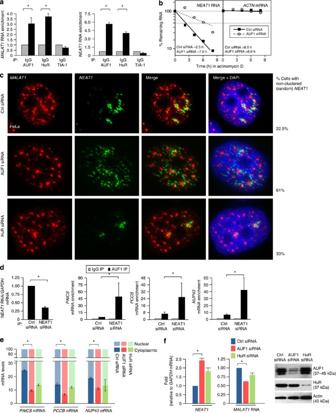Figure 3: AUF1 destabilizesNEAT1and facilitates accumulation of exported mRNAs. (a) RIP analysis was carried out to measure the relative enrichment of lncRNAsMALAT1andNEAT1, as measured by RT-qPCR analysis (after normalization toGAPDHmRNA levels) in AUF1, HuR and TIA-1 RNPs or IgG. (b) Forty-eight hours after silencing AUF1, the half-life ofNEAT1RNA was measured as explained in the Methods section. (c) FISH analysis ofNEAT1andMALAT1RNAs in HeLa cells 48 h after transfection of control, AUF1 or HuR siRNAs. DNA was counterstained with DAPI (blue). (d) Forty-eight hours after transfecting HeLa cells with control (Ctrl) or NEAT1 siRNA, RIP analysis was performed to measure the relative enrichment ofPAICS,PCCBandNUP43mRNAs (normalized toGAPDHmRNA) in AUF1 RNPs. (e) Relative distribution ofPAICS,PCCBandNUP43mRNAs in the nucleus and cytoplasm 48 h after transfection of control, AUF1 or HuR siRNA, respectively. (f) Levels ofNEAT1andMALAT1RNAs (normalized toGAPDHmRNA) 48 h after silencing HuR or AUF1 in HeLa cells. Data ina,b,d–fare the means and s.d. from three independent experiments; *P<0.05, using Student’st-test. The Cufflinks software package was used to align sequence reads to the genome and for determination of mRNA abundance ( Supplementary Table 3 ). Subsequently, we selected mRNAs robustly expressed with an intensity of more than three RPKM (reads per kilobase per million) for further analysis of mRNA abundance change after overexpression of AUF1 ( Supplementary Table 3 ). The cumulative abundance change of 3,105 AUF1 target RNAs on overexpression of the individual isoforms (the intervention used to identify AUF1 targets; Fig. 1 ) was compared with 4,529 non-targets. Comparison of the effects of overexpressing AUF1 relative to the control group (empty vector) showed that AUF1 binding was associated with reductions in target levels, in agreement with AUF1 promoting RNA decay ( Fig. 2a,b ); binning the 3,105 AUF1 targets into bins of decreasing T-to-C conversion frequency revealed similar results as binning the targets by number of binding sites ( Fig. 2c ), as targets with strongest AUF1 interactions were downregulated most efficiently. In other words, sorting the PAR-CLIP sites by frequency of T-to-C mutations helps to identify the top functional sites. In sum, our analysis indicates that AUF1 acts globally as a negative regulator of mRNA abundance. Figure 2: AUF1 lowers the levels of target mRNA subsets. ( a ) Relative overexpression of each AUF1 isoform, as assessed by RT-qPCR analysis; data are the means+s.d. from three independent experiments. ( b ) Cumulative distribution analysis in abundance of AUF1 PAR-CLIP target mRNAs after AUF1 overexpression. The red lines are almost exactly superimposed on the orange lines. ( c ) Cumulative distribution analysis of 3,105 AUF1 target mRNAs binned by target site number or T-to-C frequency. Significance in graphs in b , c was determined using the KS (Kolmogorov–Smirnov) test. Full size image The majority of AUF1 PAR-CLIP tags were found in introns; depending on the isoform, intron tags comprised 53–85% independent tags, in the range seen for HuR (59%; Supplementary Fig. 3a ; Supplementary Tables 1 and 2 ). Overexpression of each AUF1 isoform in HEK293 cells separately followed by comparison of the relative abundance of transcripts on a global scale by RNA-Seq indicated that AUF1 altered the abundance of select groups of alternative transcripts, possibly by affecting their splicing and/or stability ( Fig. 3b ; Supplementary Fig. 3c ). Figure 3: AUF1 destabilizes NEAT1 and facilitates accumulation of exported mRNAs. ( a ) RIP analysis was carried out to measure the relative enrichment of lncRNAs MALAT1 and NEAT1 , as measured by RT-qPCR analysis (after normalization to GAPDH mRNA levels) in AUF1, HuR and TIA-1 RNPs or IgG. ( b ) Forty-eight hours after silencing AUF1, the half-life of NEAT1 RNA was measured as explained in the Methods section. ( c ) FISH analysis of NEAT1 and MALAT1 RNAs in HeLa cells 48 h after transfection of control, AUF1 or HuR siRNAs. DNA was counterstained with DAPI (blue). ( d ) Forty-eight hours after transfecting HeLa cells with control (Ctrl) or NEAT1 siRNA, RIP analysis was performed to measure the relative enrichment of PAICS , PCCB and NUP43 mRNAs (normalized to GAPDH mRNA) in AUF1 RNPs. ( e ) Relative distribution of PAICS , PCCB and NUP43 mRNAs in the nucleus and cytoplasm 48 h after transfection of control, AUF1 or HuR siRNA, respectively. ( f ) Levels of NEAT1 and MALAT1 RNAs (normalized to GAPDH mRNA) 48 h after silencing HuR or AUF1 in HeLa cells. Data in a , b , d – f are the means and s.d. from three independent experiments; * P <0.05, using Student’s t -test. Full size image AUF1-dependent degradation of NEAT1 Next, we examined lncRNAs interacting with AUF1 from PAR-CLIP data sets (>1,700 lncRNAs; Supplementary Table 1 ). NEAT1 and MALAT1 were identified among the best-known target lncRNAs ( XIST and FTX were also found). The nuclear lncRNA NEAT1 functions as a structural RNA for the assembly of nuclear paraspeckles [33] , and nuclear speckle-associated MALAT1 modulates cell cycle progression by regulating the expression or pre-mRNA processing of cell cycle genes [34] . In HeLa (human cervical carcinoma) cells, which share extensively the transcriptome of HEK293 cells and express comparable AUF1 levels ( Supplementary Fig. 4 ), we confirmed the interaction of AUF1 with NEAT1 and MALAT1 by RIP analysis ( Fig. 3a ) and by in vitro binding assays ( Supplementary Fig. 5 ). Furthermore, AUF1 destabilized NEAT1 , as depletion of AUF1 using small interfering RNA (siRNA) increased NEAT1 half-life; transcript stability was measured by incubating cells with actinomycin D to block transcription and by estimating the time required to reduce NEAT1 to 50% of its initial levels, consistent with the increased steady-state levels seen by RNA-Seq (89% increased; Fig. 3b ). Analysis of the localization of NEAT1 in HeLa cells after silencing AUF1 or HuR by RNA fluorescence in situ hybridization (RNA FISH) revealed that AUF1-depleted cells showed increased numbers of paraspeckles. Control cells showed 2 or 3 paraspeckle foci, whereas paraspeckles in AUF1-depleted cells were not clustered and distributed more diffusely over the nucleus ( Fig. 3c ). Elevated cellular levels of NEAT1 or other components of paraspeckle increase the number of nuclear paraspeckles [34] , [35] . On the basis of this observation, we hypothesized that the increase in paraspeckle number observed in AUF1-depleted cells could be due to the elevated levels of NEAT1 present in these cells. Silencing AUF1 or HuR did not affect the overall distribution or levels of other nuclear-retained RNAs, including poly(A)+ RNA, U2 snRNA, MALAT1 (or its alternative splicing function) [34] , [36] and XIST (in WI-38 human fibroblasts; Fig. 3c ; Supplementary Fig. 5 ). In addition to its role as a structural scaffold of paraspeckles, NEAT1 influences the nuclear retention of several mRNAs, including A-to-I-edited mRNAs [33] . Analysis of several well-characterized NEAT1 -regulated transcripts ( PAICS , PCCB and NUP43 mRNAs) revealed that silencing NEAT1 increased the association of AUF1 with all three mRNAs ( Fig. 3d ), without altering their steady-state levels ( Supplementary Fig. 5d ). Furthermore, AUF1-silenced cells, but not HuR-silenced cells, showed specific and significant accumulation of these mRNAs in the nucleus ( Fig. 3e ; Supplementary Figure 3d ), and greater than twofold higher levels of NEAT1 RNA, in keeping with its increased stability ( Fig. 3b,f ). Taken together, our results indicate that AUF1 modulates NEAT1 levels and localization in the nucleus. Through this influence, AUF1 might control the nuclear export of a specific set of NEAT1 -target mRNAs whose localization is regulated by NEAT1 . AUF1 cooperates with HuR to control mRNA translation In light of the RREs shared between AUF1 and HuR ( Fig. 1e ; Supplementary Fig. 1 ), we hypothesized that AUF1 and HuR might jointly modulate the translation of shared target mRNAs on a transcriptome-wide scale. We used ribosome profiling [37] to identify target mRNAs potentially subject to translational control by AUF1 or HuR. In HeLa cells with normal or silenced levels of AUF1 or HuR, we digested RNA that was unprotected by ribosomes, purified monoribosomes and prepared small-RNA libraries for high-throughput sequencing ( Fig. 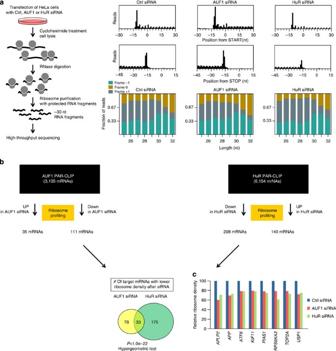Figure 4: AUF1 and HuR share common target mRNAs for translation control. (a) Left, schematic of ribosome profiling after silencing AUF1 or HuR in HeLa cells. Right top, graphs summarize ribosome densities near the start and stop codons (meta-gene average). Right bottom, trinucleotide periodicity with framing information for footprints that fall within protein-coding genes. (b) Comparison of shared target AUF1 and HuR target mRNAs subject to translation control. (c) Relative ribosome density on representative mRNAs after AUF1 or HuR silencing. 4a ; Supplementary Table 4 ). Ribosome densities near start/stop codons and trinucleotide periodicity ( Fig. 4a ) provided confidence that the ribosome profiling yielded similar patterns of ribosome occupancy as those reported previously. Figure 4: AUF1 and HuR share common target mRNAs for translation control. ( a ) Left, schematic of ribosome profiling after silencing AUF1 or HuR in HeLa cells. Right top, graphs summarize ribosome densities near the start and stop codons (meta-gene average). Right bottom, trinucleotide periodicity with framing information for footprints that fall within protein-coding genes. ( b ) Comparison of shared target AUF1 and HuR target mRNAs subject to translation control. ( c ) Relative ribosome density on representative mRNAs after AUF1 or HuR silencing. Full size image Ribosome profiling identified 116 mRNAs showing increased (>20%) ribosome densities after AUF1 silencing, while 231 mRNAs showed decreased ribosome densities (<20%). Among these mRNAs, >30% had AUF1 PAR-CLIP tags (111 mRNAs; Supplementary Table 4 ), suggesting that these mRNAs were candidates for direct translational control by AUF1, and most of them (69.8%) did not show altered abundance after silencing AUF1. We also identified 140 and 208 mRNAs whose ribosome densities increased or decreased after HuR silencing and had HuR PAR-CLIP tags. Interestingly, among the HuR and AUF1 translation targets, 33 mRNAs showed decreased ribosome density after silencing AUF1 or HuR, supporting the view that AUF1 and HuR jointly modulated common target mRNAs for translation activation, while only 9 mRNAs showed increased ribosome density after silencing AUF1 or HuR (data not shown), indicating that the two RBPs mainly co-stimulate target mRNA translation ( Fig. 4b ). One of the candidate mRNAs for translational control by both AUF1 and HuR encodes the topoisomerase subunit 2a (TOP2A). Ribosome profiling revealed that the ribosome density on TOP2A mRNA decreased >20% after silencing AUF1 or HuR ( Fig. 4c ). Since we previously reported that HuR activates TOP2A mRNA translation by competing with miR-548c-3p [38] , we tested whether AUF1 similarly affected TOP2A mRNA translation. Interaction of AUF1 and TOP2A mRNA was confirmed by RIP analysis; furthermore, AUF1 silencing decreased TOP2A protein level, whereas AUF1 overexpression increased TOP2A protein level without changes in TOP2A mRNA levels ( Fig. 6a,b ). Luciferase reporter and RIP assays supported the notion that AUF1 elicited its regulation via the TOP2A 3′UTR ( Fig. 6c,d ). Figure 6: In vitro analysis of AUF1 and HuR binding to target mRNAs and regulation of translation. 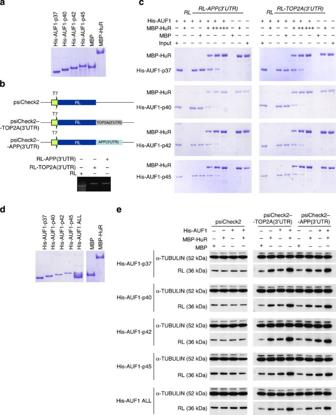Figure 6:In vitroanalysis of AUF1 and HuR binding to target mRNAs and regulation of translation. (a–c) Recombinant His-AUF1, MBP and MBP-HuR proteins (a) and templates forin vitrotranscription of substrate RNAs, as well as transcribed RNA (b, bottom) used in biotin pull-down assays (c). Biotin pulldown was carried out usingRL,RL-APP(3′UTR)orRL-TOP2A(3′UTR)(1 μg each) in the presence of 1 μg of recombinant His-AUF1 and 0, 2, 4 or 6 μg MBP-HuR before pulldown using streptavidin sepharose beads. Following SDS–PAGE, proteins were visualized by staining with Coomassie blue. (d,e) Individual and combined (ALL) recombinant proteins (d) were used inin vitrotranslation assays. Rabbit reticulocyte lysate reactions contained T7 RNA polymerase, 0.5 μg of the plasmids inb, expressing reporterRL,RL-APP(3′UTR)orRL-TOP2A(3′UTR)mRNAs, 0.5 μg of recombinant protein (His-AUF1 alone or in combination, MBP-HuR or MBP). Reaction components were separated with SDS–PAGE and western blot analysis was performed to detect Renilla luciferase (RL) and loading control α-Tubulin. Data are representative of three independent experiments. ( a – c ) Recombinant His-AUF1, MBP and MBP-HuR proteins ( a ) and templates for in vitro transcription of substrate RNAs, as well as transcribed RNA ( b , bottom) used in biotin pull-down assays ( c ). Biotin pulldown was carried out using RL , RL-APP(3′UTR) or RL-TOP2A(3′UTR) (1 μg each) in the presence of 1 μg of recombinant His-AUF1 and 0, 2, 4 or 6 μg MBP-HuR before pulldown using streptavidin sepharose beads. Following SDS–PAGE, proteins were visualized by staining with Coomassie blue. ( d , e ) Individual and combined (ALL) recombinant proteins ( d ) were used in in vitro translation assays. Rabbit reticulocyte lysate reactions contained T7 RNA polymerase, 0.5 μg of the plasmids in b , expressing reporter RL , RL-APP(3′UTR) or RL-TOP2A(3′UTR) mRNAs, 0.5 μg of recombinant protein (His-AUF1 alone or in combination, MBP-HuR or MBP). Reaction components were separated with SDS–PAGE and western blot analysis was performed to detect Renilla luciferase (RL) and loading control α-Tubulin. Data are representative of three independent experiments. Full size image In keeping with the lower ribosome density of TOP2A mRNA after silencing AUF1 or HuR in HeLa cells, fractionation of polysomes through sucrose gradients ( Fig. 5a ) revealed that, while silencing AUF1 or HuR did not affect total TOP2A mRNA levels ( Fig. 5b ) or their stability (ref. 38 , data not shown), the distribution of TOP2A mRNA shifted towards smaller ribosome fractions ( Fig. 5c ), in agreement with the lower ribosome density of TOP2A mRNA seen after silencing AUF1 or HuR ( Fig. 4b ). In addition, simultaneous AUF1 and HuR silencing shifted the distribution of TOP2A mRNA in polysomes further towards non-translating fractions of the gradient, devoid of ribosomal components ( Fig. 5c ). We observed similar changes in APP mRNA and USP1 mRNA translation without changes in the steady-state levels of these mRNAs ( Fig. 5b,c ). These changes were reflected in the levels of TOP2A, USP1 and APP proteins by western blot analysis ( Fig. 5d ). 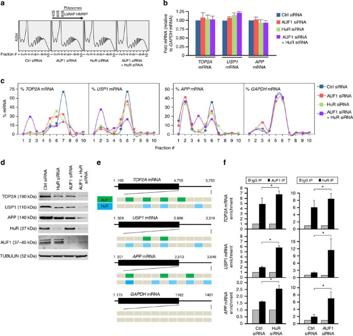These results demonstrate that AUF1 can cooperate with HuR in the translational activation of target mRNAs. Figure 5: AUF1 cooperates with HuR for mRNA translation. (a–d) Forty-eight hours after HeLa cells were transfected with the siRNAs indicated, lysates were fractionated through sucrose gradients (a); arrow indicates the direction of sedimentation; −, fractions without ribosomal components, 40S and 60S, small and large ribosome subunits, respectively; 80S, monosome; LMWP and HMWP, low- and high-molecular weight polysomes, respectively. The relative total levels ofTOP2A, APP, USP1mRNAs (normalized toGAPDHmRNA) were assessed (b) and the distribution (%) ofTOP2A, APP, USP1mRNAs and controlGAPDHmRNA was measured by RT-qPCR analysis of RNA in each of 10 gradient fractions (c) and the levels of the encoded proteins in whole-cell lysates were assessed by western blot analysis (d). (e) Schematic of AUF1- and HuR-binding sites on the 3′UTRs ofTOP2A, APP, USP1mRNAs and controlGAPDHmRNA. (f) Forty-eight hours after silencing HuR or AUF1, the levels ofTOP2A, APP, USP1mRNAs in AUF1 IP or HuR IP were measured by RIP followed by RT-qPCR analysis; data were normalized to controlGAPDHmRNA levels in each IP. Data inb,fare the means and s.d. from three independent experiments; *P<0.05, Student’st-test. Figure 5: AUF1 cooperates with HuR for mRNA translation. ( a – d ) Forty-eight hours after HeLa cells were transfected with the siRNAs indicated, lysates were fractionated through sucrose gradients ( a ); arrow indicates the direction of sedimentation; −, fractions without ribosomal components, 40S and 60S, small and large ribosome subunits, respectively; 80S, monosome; LMWP and HMWP, low- and high-molecular weight polysomes, respectively. The relative total levels of TOP2A, APP, USP1 mRNAs (normalized to GAPDH mRNA) were assessed ( b ) and the distribution (%) of TOP2A, APP, USP1 mRNAs and control GAPDH mRNA was measured by RT-qPCR analysis of RNA in each of 10 gradient fractions ( c ) and the levels of the encoded proteins in whole-cell lysates were assessed by western blot analysis ( d ). ( e ) Schematic of AUF1- and HuR-binding sites on the 3′UTRs of TOP2A, APP, USP1 mRNAs and control GAPDH mRNA. ( f ) Forty-eight hours after silencing HuR or AUF1, the levels of TOP2A, APP, USP1 mRNAs in AUF1 IP or HuR IP were measured by RIP followed by RT-qPCR analysis; data were normalized to control GAPDH mRNA levels in each IP. Data in b , f are the means and s.d. from three independent experiments; * P <0.05, Student’s t -test. Full size image Further investigation indicated that AUF1 and HuR bound on two shared sites on the TOP2A 3′UTR ( Fig. 5e ). We identified similar overlapping binding sites for AUF1 and HuR on APP and USP1 mRNAs. To test whether these interactions were cooperative or competitive, we performed RIP analysis of HuR or AUF1 after silencing AUF1 or HuR, respectively. As shown, HuR silencing promoted the interaction of AUF1 with target TOP2A , APP and USP1 mRNAs, while AUF1 silencing increased the binding of HuR to these mRNAs ( Fig. 5f ); when both AUF1 and HuR were silenced simultaneously, neither RBP associated with any of these mRNAs ( Supplementary Fig. 5g ). These results indicate that AUF1 may compete with HuR for binding to individual target 3′UTRs, even though AUF1 and HuR jointly promote their translation, likely because there are multiple sites of interaction. Taken together, we propose that the combined influence of HuR and AUF1 on some target mRNAs is essential for their translation. AUF1 and HuR share targets and regulate translation in vitro We sought additional support for the joint influence of AUF1 and HuR on target RNAs using in vitro approaches. First, we investigated the binding of recombinant AUF1 (His-AUF1) and HuR (MBP-HuR) ( Fig. 6a ) to several biotinylated reporter mRNAs: renilla luciferase ( RL ) mRNA (expressed from parent control plasmid psiCheck2), RL-TOP2A(3 ′ UTR) mRNA (expressed from psiCheck2-TOP2A(3′UTR)) and RL-APP(3′UTR) mRNA (expressed from psiCheck2-APP(3′UTR)); in each case, expression of the reporter RNA was driven by the T7 RNA polymerase promoter ( Fig. 6b ). Biotinylated RL , RL-TOP2A(3′UTR) and RL-APP(3′UTR) were incubated with 1 μg of each recombinant His-AUF1 isoform in the presence of 0, 2, 4 or 6 μg MBP-HuR; following pulldown of biotinylated RNA using streptavidin beads, the bound proteins were separated by SDS–polyacrylamide gel electrophoresis (PAGE) and detected using Coomassie stain ( Fig. 6c ). These data revealed that HuR was capable of competing with AUF1 for binding to these shared target RNAs. The relative influence of AUF1 and HuR on translation of these RNAs was also tested in vitro using the same recombinant proteins (His-AUF1 and MBP-HuR; Fig. 6d ) added to rabbit reticulocyte lysates containing the plasmids shown in Fig. 6b , which expressed RL , RL-TOP2A(3′UTR) and RL-APP(3′UTR) mRNAs driven by T7 RNA polymerase. Forty minutes later, reaction mixtures were size separated by SDS–PAGE and the newly synthesized Renilla luciferase detected by western blot analysis. As shown in Fig. 6e , translation of luciferase from psiCheck2 (expressing RL mRNA) was not affected by HuR or AUF1 levels; by contrast, translation of luciferase from RL-TOP2A(3′UTR) mRNA (from psiCheck2-TOP2A(3′UTR)) or from RL-APP(3′UTR) mRNA (from psiCheck2-APP(3′UTR)) was enhanced by the presence of HuR or AUF1 and was further enhanced when both RBPs were added together. Together, these data support the results in Fig. 5d that AUF1 and HuR can compete for binding and cooperate in the translational activation of shared target mRNAs. AUF1 prevents subset mRNA decay and protects DNA Interestingly, the effect of AUF1 on mRNA abundance by AUF1 in HEK293 cells was tightly dependent on the levels of both AUF1 and the target mRNAs. While overexpression of AUF1 from plasmids led to AUF1 target destabilization ( Fig. 2a ), silencing AUF1 in HEK293 also reduced the levels of several AUF1 targets ( Fig. 7a ; Supplementary Table 5 ; Supplementary Note ). However, the magnitude of the effect on individual target mRNAs was different and the mRNAs which changed most strongly in the overexpression data set did not overlap extensively with mRNAs changed in the silencing data set: among 423 target mRNAs downregulated after AUF1 overexpression (greater than twofold change), only 28 mRNAs overlapped with the silencing data sets. The effect of endogenous AUF1 protein on mRNA abundance varied somewhat depending on the cell type, as AUF1 silencing in WI-38 cells lowered AUF1 mRNA target levels dependent on the extent of AUF1 interaction ( Fig. 7b ; Supplementary Table 6 ). As expected, given the known mRNA-stabilizing effect of HuR, its knockdown in WI-38 cells led to decreased AUF1 target mRNA levels ( Fig. 7c ; Supplementary Table 6 ). Interestingly, AUF1 target mRNAs were also reduced in senescent fibroblasts (population doubling (PDL) 55 compared with PDL 15), when AUF1 levels are lower [39] ( Fig. 7d ; Supplementary Table 6 ). These results suggest that AUF1 can function in target mRNA upregulation, not only downregulation; in this regard, it is important to note that some mRNAs could be positively regulated through AUF1-driven transcription (as reported [40] , [41] and discussed below). 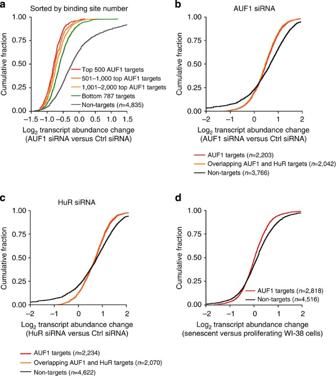Figure 7: AUF1 stabilizes target mRNAs globally. (a) Cumulative distribution analysis of 4,835 AUF1 target mRNAs binned by target site number in HEK293 cells. (b,c) In WI-38 cells, cumulative distribution analysis of the abundance of AUF1 PAR-CLIP target mRNAs after silencing AUF1 (b) or HuR (c). (d) Cumulative distribution analysis of AUF1 target mRNAs in senescent (PDL 55) and proliferating (PDL 15) WI-38 cells. Figure 7: AUF1 stabilizes target mRNAs globally. ( a ) Cumulative distribution analysis of 4,835 AUF1 target mRNAs binned by target site number in HEK293 cells. ( b , c ) In WI-38 cells, cumulative distribution analysis of the abundance of AUF1 PAR-CLIP target mRNAs after silencing AUF1 ( b ) or HuR ( c ). ( d ) Cumulative distribution analysis of AUF1 target mRNAs in senescent (PDL 55) and proliferating (PDL 15) WI-38 cells. Full size image AUF1 potently inhibits cellular senescence and delays the aging phenotype [16] , [39] . Although AUF1 lowers p16 mRNA stability and increases transcription of the TERT mRNA, encoding telomerase, the full set of specific mediators of this influence have not been identified. A comparison of the AUF1 PAR-CLIP data set and whole-cell mRNA-Seq after silencing AUF1 in WI-38 human diploid fibroblasts identified numerous AUF1 target mRNAs altered with senescence: 285 were upregulated and 219 were downregulated ( Fig. 8a ). A subsequent comparison of RNA-Seq data sets from proliferating (early-passage) and senescent (late-passage) WI-38 cells further identified 43 mRNAs whose levels increased (twofold cutoff) in senescent cells in an AUF1-dependent manner and 69 mRNAs downregulated (fivefold cutoff) in senescent cells. A similar analysis was performed with HuR PAR-CLIP to identify common mRNA targets of AUF1 and HuR in stability control during senescence ( Fig. 8a ). 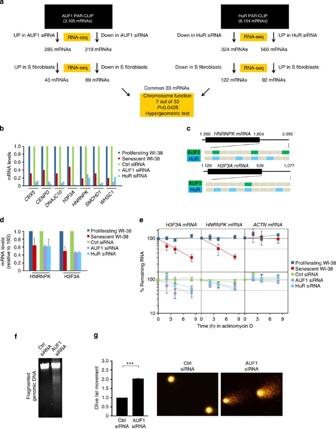Figure 8: AUF1 protects cells from DNA damage. (a) AUF1 and HuR target mRNAs downregulated (as determined by RNA-Seq) in senescent (S) WI-38 human diploid fibroblasts. (b) Relative expression (as assessed by RNA-Seq) of target mRNAs in proliferating and senescent fibroblasts, as well as in proliferating WI-38 cells after transfection of control, AUF1 or HuR siRNAs. (c) Schematic of AUF1- and HuR-binding sites onHNRNPKandH3F3AmRNAs. (d,e) Cells prepared as described inbwere used for assessment of steady-state levels using RT-qPCR (d) and relative stability (e) ofHNRNPKandH3F3AmRNAs; mRNA levels and half-lives were calculated as described inFig. 3b; data are the means and s.d. from three independent experiments. (f,g) DNA fragmentation assay (f) and comet assay (g) were performed after transfection of HeLa cells with control (Ctrl) siRNA or AUF1 siRNA. ***P<0.001. Figure 8: AUF1 protects cells from DNA damage. ( a ) AUF1 and HuR target mRNAs downregulated (as determined by RNA-Seq) in senescent (S) WI-38 human diploid fibroblasts. ( b ) Relative expression (as assessed by RNA-Seq) of target mRNAs in proliferating and senescent fibroblasts, as well as in proliferating WI-38 cells after transfection of control, AUF1 or HuR siRNAs. ( c ) Schematic of AUF1- and HuR-binding sites on HNRNPK and H3F3A mRNAs. ( d , e ) Cells prepared as described in b were used for assessment of steady-state levels using RT-qPCR ( d ) and relative stability ( e ) of HNRNPK and H3F3A mRNAs; mRNA levels and half-lives were calculated as described in Fig. 3b ; data are the means and s.d. from three independent experiments. ( f , g ) DNA fragmentation assay ( f ) and comet assay ( g ) were performed after transfection of HeLa cells with control (Ctrl) siRNA or AUF1 siRNA. *** P <0.001. Full size image Comparison of PAR-CLIP and RNA-Seq data suggested that 33 shared mRNAs were both AUF1 and HuR targets and declined during senescence ( Fig. 8a ). Interestingly, 7 among the 33 ( CBX5 , CENPD , DNAJC10 , H3F3A , HNRNPK , SMCHD1 and WHSC1 mRNAs) encoded proteins HP1α, centromere protein D, DNAJ, H3F3A, hnRNPK, SMCHD1 (structural maintenance of chromosomes flexible hinge domain 1) and WHSC1/NSD2 (histone–lysine N -methyltransferase NSD2), which are closely involved in preserving chromosome function. These mRNAs, as measured by RNA-Seq, were less abundant in senescent WI-38 cells, as well as after silencing HuR or AUF1 in WI-38 cells ( Fig. 8b ), suggesting that AUF1 and HuR might help maintain genomic stability. In addition, HNRNPK and H3F3A mRNAs contain overlapping AUF1 and HuR PAR-CLIP tags ( Fig. 8c ); indeed, their levels and half-lives were lower when HuR or AUF1 were silenced ( Fig. 8d,e ). The variability in ‘fold’ changes arises from the different detection methods used (RNA-Seq in Fig. 8b and reverse transcription-quantitative PCR (RT-qPCR) in Fig. 8d ). Finally, since TOP2A, USP1, APP, hnRNPK, SMCHD1 and H3F3a are DNA damage response proteins, we assessed the extent of general DNA damage after AUF1 silencing. As shown, AUF1 silencing led to more genomic DNA fragmentation ( Fig. 8f ) and increased DNA damage as measured by single-cell gel electrophoresis (comet) assays ( Fig. 8g ). Taken together, our results indicate that AUF1, through its influence on target mRNAs, helps to protect cells from DNA damage. Numerous AUF1 RNPs have been studied using a number of in vitro and in vivo methods. These reports have shown primarily that AUF1 binds AU-rich RNAs and promotes their decay. However, there are significant biases in these earlier analyses. Analyses to identify AUF1 binding to tagged RNAs (for example, radiolabeled, biotinylated, fluorescent) required that the target RNAs be chosen a priori , while traditional methods to study endogenous AUF1 and endogenous RNAs, like RIP chip [25] , only identified mRNAs detectable by the microarray and did not inform about the specific site of interaction. Although the method used here, PAR-CLIP, also has limitations, as it is lengthy, requires substantive bioinformatic expertise, and carries some bias associated with the ligation of adapters to the recovered RNA using RNA ligases [27] , [42] , it provides a much more complete account of both the identity of AUF1 target transcripts (mRNAs and ncRNAs) and the sequences at the specific sites where AUF1 interacts. The characteristic T-to-C mutation, which allows the pinpointing of sites of interaction between RBPs and RNA in PAR-CLIP, occurs at a high frequency (it is present at >50% of sequence reads at a high-quality site) and allows for a very efficient separation of noise from background sequences. Thus, combined with available and user-friendly software tools (for example, PIPE-CLIP, PARalyzer, CLIPZ, doRiNA), T-to-C mutations permit the detection of high-quality RBP-binding sites and may provide a qualitative measure of functional RBP–RNA interactions. The AUF1 PAR-CLIP libraries have yielded some surprising and important discoveries. First, the preferred sites were not AU-rich, but were instead U-, GU- and UG-rich ( Fig. 1d ); the four isoforms did not overlap exactly in their preferred sites, with AUF1 p45 showing the closest RNA target site preference to that of HuR ( Fig. 1d ; Supplementary Fig. 1f ). Second, AUF1 binds numerous lncRNAs ( Supplementary Table 1 ). Binding of AUF1 to lncRNA NEAT1 was associated with decreased NEAT1 stability and with the increased nuclear accumulation of NEAT1 -exported mRNAs ( Fig. 3 ). This evidence points to AUF1 as a possible indirect regulator of mRNA export. The influence of AUF1 on the levels of other lncRNAs and possibly on the export of other mRNAs remains to be studied systematically. In addition, since different AUF1 isoforms can oligmerize with other AUF1 isoforms [12] , each PAR-CLIP library reflects the RNA with which one tagged AUF1 binds, whether as a monomer or by oligmerizing with other AUF1 isoforms. We employed PAR-CLIP to gain information on AUF1 through integration with other data sets. Joint analysis of AUF1 PAR-CLIP with RNA-Seq after AUF1 overexpressing and silencing, yielded global information about the role of AUF1 on steady-state levels of AUF1 target transcripts. These results ( Fig. 2 ) revealed that AUF1 robustly reduced the steady-state levels of many target RNAs, agreeing with the mRNA decay-promoting function of AUF1 that we and others have reported [11] , [12] , [24] , [30] , [43] , but possibly also reflecting the recently identified role of AUF1 in transcriptional control, as discussed below. Measurement of NEAT1 half-life ( Fig. 3b ) revealed that AUF1 was also capable of lowering the steady-state levels of lncRNAs. The mechanisms whereby AUF1 reduces the stability of target transcripts are not fully known, but they may be associated with the recruitment by AUF1 of the exosome or the proteasome [44] , [45] or, as shown in a recent high-throughput analysis of AUF1 target mRNAs, by competition or cooperation with microRNAs [46] . Contrary to expectation, a subset of AUF1 targets was found to be positively regulated by AUF1: 174 mRNAs were upregulated after AUF1 overexpression, while 75 mRNAs were downregulated after AUF1 silencing ( Supplementary Tables 3 and 5 ). Some AUF1 target mRNAs have already been reported to be stabilized by AUF1, including PTH , VHL and MAT1A mRNAs [18] , [19] , [47] . It is possible that AUF1 elicits this influence by competing with other, perhaps more potent, decay-promoting RBPs or with microRNAs or other ncRNAs, which bind the same mRNA sequences, although such factors have not been identified systematically. These results indicate that the global impact of an RBP on target RNAs must be studied using unbiased methods such as PAR-CLIP combined with RNA-Seq analyses. In this regard, it must also be mentioned that AUF1 was reported to enhance the transcription of MYC , CD21 and telomerase ( TERT ) genes [16] , [40] , [41] . The AUF1 target DNA sequence is not known, but global analysis of AUF1 chromatin IP (ChIP) coupled with global run-on sequencing (GRO-seq) analysis will be a helpful approach to elucidate systematically the role of AUF1 on transcription. It will be particularly interesting to investigate whether AUF1 can transcriptionally upregulate the same mRNAs whose stability it can modulate. Integration of AUF1 PAR-CLIP with differential RNA expression profile using RNA-Seq indicated that AUF1 binding, which was most frequently observed at intron sites, was associated with the exclusion and inclusion of different introns ( Supplementary Fig. 3c ). In earlier global studies, AUF1 was shown to associate with pre-mRNA [25] , [48] , but to our knowledge this is the first indication that AUF1 could modulate alternative splicing. Studies are underway to investigate this function in depth. Integration of PAR-CLIP with ribosome profiling provided novel insight into the function of AUF1 as regulator of translation. It revealed that AUF1 affected the translation status of a number of target mRNAs: while AUF1 reduced the polysome sizes of a small subset of target mRNAs, it enhanced the translation of a larger subset of targets ( Fig. 4b ), as silencing AUF1 lowered polysomes sizes by >20%. An earlier report showed that AUF1 promoted the translation of MYC mRNA by displacing the translational repressor TIAR [21] ; while AUF1 also promoted translation of CD83 mRNA, the mechanism has not been elucidated [49] . However, AUF1 formed strong interactions with eIF4G and poly(A)-binding protein, thereby possibly enhancing the translation of a subset of mRNAs [20] . The promotion of translation by AUF1 was confirmed in vitro for APP 3′UTR and TOP2A 3′UTR ( Fig. 6 ), and was further enhanced by the presence of HuR. Whether the translational effects of AUF1 are generally tied to the actions (for example, competition or cooperation) of other RBPs or ncRNAs warrants further analysis. Finally, the fact that many AUF1 target mRNAs do not appear to be regulated at the level of steady-state abundance or translational engagement suggests that AUF1 may control other steps in RNA metabolism (for example, mRNA transport or storage) or that AUF1 influence on some target mRNAs may only be revealed when cells are stimulated (for example, through the actions of mitogenic, immune or stress agents). AUF1 deficiency caused accelerated aging in mice and enhanced senescence in mouse and human cells [16] , [39] . Here, the impact of AUF1 targets identified by PAR-CLIP and AUF1 function, as assessed via other high-throughput methods (for example, RNA-Seq, other PAR-CLIP data sets, ribosome profiling), were probed in the context of cellular senescence. Several AUF1 target mRNAs encoding well-established genotoxic stress–response proteins (TOP2A, USP1, APP, hnRNPK, SMCHD1 and H3F3A) were under positive regulation by AUF1. In agreement with this influence, we observed enhanced DNA damage after AUF1 silencing, both by monitoring genomic DNA fragmentation and by comet assays ( Fig. 8f,g ). Since damaged DNA accumulates with aging and some genetic DNA repair defects that can resemble premature aging [49] , the reduced DNA repair in the presence of low AUF1 explains at least in part the enhanced aging observed in AUF1-deficient mice [16] . Closely related to DNA damage are two other underlying defects in aging: aberrant patterns of expressed transcripts and altered chromatin structure and epigenetic modifications. The present studies serve as a platform for further analysis of AUF1 in these molecular mechanisms, as we strive to understand better the complexity of AUF1 actions in processes such as aging and cancer. Cell culture, transfection, siRNAs and plasmids Human embryonic kidney 293 (HEK293) cells, HeLa cells and diploid lung (WI-38) fibroblasts were cultured in DMEM (Invitrogen) supplemented with 10% (v/v) fetal bovine serum and antibiotics. Cells were transfected (Lipofectamine 2000, Invitrogen) with control siRNA (5′-UUCUCCGAACGUGUCACGUdTdT-3′), AUF1 siRNA (5′-AAGAUCCUAUCACAGGGCGATdTdT-3′), HuR siRNA (5′-CGUAAGUUAUUUCCUUUAAdTdT-3′), and NEAT1 siRNA [33] , each at 20 nM. Plasmids expressing AUF1 were described [50] and were transfected at 50 ng ml −1 (pEGFP, pEGFP-TOP2A(3′)) or at 1–2 μg ml −1 (pcDNA, pcDNA-AUF1). TOP2A 3′UTR reporter constructs were made by inserting TOP2A 3′UTR into pEGFP-C1. Transfected cells were typically analysed 48 h later. Comet assays were performed using established protocols [51] . PAR-CLIP analysis For AUF1 PAR-CLIP [27] , [52] , the four isoforms of AUF1 (p37, p40, p42 and p45) tagged with a Flag epitope [50] were expressed in HEK293 cells. One hundred million cells per culture were incubated in medium supplemented with 100 μM 4SU for 16 h, washed with phosphate-buffered saline and irradiated with 0.15 mJ cm −2 , 365 nm ultraviolet light in a Spectrolinker XL-1500 UV crosslinker to crosslink RNA to AUF1, and harvested and lysed in the equivalent of three cell pellet volumes of NP-40 lysis buffer. The cleared cell lysates were treated with 1 U μl −1 RNase T1 (Fermentas) and AUF1 proteins immunoprecipitated with monoclonal anti-FLAG antibodies (M2, Sigma) bound to Protein G Dynabeads. The RNA residing in the immunoprecipitate was further trimmed with 100 U ml −1 RNase T1. The beads were washed in lysis buffer and resuspended in one bead volume of dephosphorylation buffer. RNA was dephosphorylated and radioactively labelled with [γ- 32 P]-ATP. The protein–RNA complexes were separated by SDS–PAGE, and RNA–protein complexes visualized by autoradiography. The radioactive bands migrating at ~37, 40, 42 and 45 kDa were recovered and the protein–RNA complex was electroeluted from the gel. The protein was removed by digestion in proteinase K buffer in the presence of 0.2 mg ml −1 proteinase K (Roche). The RNA was then recovered by acidic phenol/chloroform extraction and ethanol precipitation, converted into a cDNA library and sequenced using an Illumina platform. Processed reads were aligned to the reference genome (GRCh37/hg19) by the Bowtie algorithm (0.12.7), allowing for two alignment errors (mutation, insertion or deletion). For each read, only the best mapping was reported out of a maximum of 10 genomic matches. Any tag with over 10 genomic matches were discarded. After the conversion subtraction, reads that mapped to only one genomic location were retained for further analysis. For analysis, the PARalyzer settings were set to require a minimum of five sequence reads per group and allow a maximum of one mismatch per sequence read. A PARalyzer-defined group was considered a binding site only if it had a T-to-C mutation rate of 0.25, contained more than five sequence reads with T-to-C conversions and had two or more distinct crosslinking sites. To approximate binding intensity using crosslinked read frequencies, raw sequence reads (rather than non-redundant sequence reads) were counted. The problem of PCR amplification bias was avoided by limiting the number of PCR cycles used for cDNA amplification to stay within the exponential amplification phase of the PCR reaction. Measurement of RNA stability To measure RNA stability, cells were treated with actinomycin D (2.5 μg ml −1 ) for varying time periods whereupon total RNA was extracted and measured by RT-qPCR analysis to determine their half-life (( t 1/2 ), the time needed for each transcript to reach 50% of their original abundance). Transcript levels were normalized to the abundance of 18S rRNA. Subcellular fractionation Cytosolic and nuclear fractions were collected after lysing cells with a buffer containing 10 mM Tris-HCl, pH 7.4, 100 mM NaCl, 2.5 mM MgCl 2 and 40 μg ml −1 digitonin for 10 min and centrifuging the resulting lysates at 2,060 g for 10 min at 4 °C. The supernatant was used for the cytosolic fraction. The pellets were washed, incubated with RIPA buffer at 4 °C for 10 min and the nuclear fraction collected after centrifugation at 4 °C for 10 min at 21,000 g . Western blot analysis and polysome assays Whole-cell lysates, prepared in RIPA buffer, were separated by SDS–PAGE and transferred onto polyvinylidene difluoride membranes (Invitrogen iBlot Stack). Primary antibodies recognizing α-TUBULIN, ACTIN, TOP2A, APP and HuR were from Santa Cruz Biotechnology. Antibodies recognizing AUF1 and renilla luciferase were from Millipore. The antibody recognizing USP1 was from Abcam. HRP-conjugated secondary antibodies were from GE Healthcare. For polyribosome fractionation assays, cells were incubated with cycloheximide (Calbiochem; 100 μg ml −1 , 15 min) and cytoplasmic lysates (500 μl) isolated in polysome extraction buffer containing 20 mM Tris-HCl at pH 7.5, 100 mM KCl, 5 mM MgCl 2 , 100 μg ml −1 cycloheximide, 0.5% NP-40, and protease and RNAse inhibitors were fractionated by centrifugation through 10–50% linear sucrose gradients and divided into 10 fractions for RT-qPCR analysis to determine the distribution of TOP2A, USP1, APP and GAPDH mRNAs. RNP analysis For IP of endogenous RNP complexes (RIP analysis) from whole-cell extracts [53] , cells were lysed in 20 mM Tris-HCl at pH 7.5, 100 mM KCl, 5 mM MgCl 2 and 0.5% NP-40 for 10 min on ice and centrifuged at 10,000 g for 15 min at 4 °C. The supernatants were incubated with protein A-Sepharose beads coated with antibodies that recognized HuR (Santa Cruz Biotechnology) or AUF1 (Millipore), or with control IgG (Santa Cruz Biotechnology) for 1 h at 4 °C. After the beads were washed with NT2 buffer (50 mM Tris–HCl at pH 7.5, 150 mM NaCl, 1 mM MgCl 2 and 0.05% NP-40), the complexes were incubated with 20 U of RNase-free DNase I (15 min at 37 °C) and further incubated with 0.1% SDS and 0.5 mg ml −1 Proteinase K (15 min at 55 °C) to remove DNA or proteins, respectively. RT-qPCR analysis of the RNA isolated from the IP material was further assessed by using the primers listed ( Supplementary Table 7 ). Normalization of RIP results was carried out by quantifying in parallel the relative levels of GAPDH mRNA in each IP sample; these abundant RNAs are nonspecific contaminants present in the IP components (for example, microfuge tube, antibodies, beads). RNA FISH For RNA FISH to detect MALAT1 , NEAT1 , U2 snRNA, poly(A)+ RNA and XIST RNA, HeLa or WI-38 cells transfected with control, AUF1 or HuR siRNA-treated HeLa or WI-38 cells were cultured in six-well plates containing coverslips and fixed in 4% formaldehyde in phosphate-buffered saline (pH 7.4) for 15 min at room temperature. Hybridization was performed using either nick-translated partial cDNA probes ( MALAT1 , NEAT1 and XIST , Abbott Molecular, Des Plaines, IL) or fluorescently tagged oligonucleotide probes (for U2 snRNA and oligo dT probe for detecting poly (A) + RNA) in a moist chamber at 37 °C for 12 h. The DNA was counterstained with DAPI (4′,6-diamidino-2-phenylindole). Fluorescence images were acquired using a DeltaVision RT (Olympus, × 60, 1.42 numerical aperture oil objective; Applied Precision, Issaquah, WA) microscope. Images were collected as vertical z -stacks covering the entire nucleus and were processed using SoftWorx (DeltaVision) software. Ribosome profiling Forty-eight hours after transfecting control siRNA, AUF1 siRNA or HuR siRNA, cell lysates were incubated with RNase A/T1 mix and subjected to ultracentrifugation for ribosome preparation. From the resulting ribosome pellets, small RNAs were prepared, dephosphorylated, ligated with linker RNAs and reverse transcribed for small cDNA library preparation [54] . RNA analysis: RT-qPCR and RNA-Seq From cytosolic and nuclear fractions, Trizol (Invitrogen) was used to prepare total RNA and acidic phenol (Ambion) was used to extract RNA for RIP analysis. RT was performed using random hexamers and reverse transcriptase (Maxima, Thermo Scientific) and real-time qPCR using gene-specific primers ( Supplementary Table 7 ) and SYBR green master mix (Kapa Biosystems), using an Applied Biosystems 7300 instrument. Total RNA-Seq was carried out as explained in the Methods section, using an Illumina GA-II instrument. All of the RNA-Seq data are available at GSE52977. For RNA-Seq, total RNA quality and quantity was assessed using the Agilent 2100-Bioanalyzer; 100 ng of RNA was used for first-strand and second-strand cDNA synthesis followed by single-primer isothermal amplification using NuGEN Ovation RNA-Seq System V2 kits according to the manufacturer’s protocol. The kit amplified both polyA-tailed and non-polyA-tailed RNA and removed ribosomal RNA. The amplified cDNA was sheared using Bioruptor (Diagenode) to an average size of 250–450 bases. The sequencing library was prepared using Illumina ChIp-Seq kits according to the manufacturer’s protocol (Illumina, San Diego, CA). In short, the ends of the fragments were repaired using T4 DNA polymerase, E. coli DNA Pol I large fragment (Klenow polymerase) and T4 polynucleotide kinase, and adenines were added to the 3′ end. Adapters were ligated to the DNA fragments, which were size selected (250–300 bases) after electrophoresis through a 4% agarose gel. Eighteen cycles of PCR amplification was performed, followed by cluster generation and sequencing with Illumina Genome Analyzer (GA-II). Sequencing was performed for 42 cycles and the images generated were analysed with the Firecrest program followed by base calls using the Bustard program; Firecrest and Bustard are part of the Illumina Analysis Pipeline package. For RNA-Seq analysis, the quality of the bases was checked using FASTQC program and called bases were aligned to the human HG19 genome using the Tophat program, the Bowtie algorithm and Ensembl hg19 (v62) as gene model annotations followed by genomic mapping. The aligned reads were assembled into transcripts (both known and novel) using Cufflinks program with Ensembl hg19 (v62) transcripts as a guide. FPKM (fragments per kilobase of exon model per million mapped reads) values were calculated after fragment bias correction and normalization to total hits. Significant changes in transcript expression levels were calculated using Cuffdiff program with a cutoff of false discovery rate <0.1 and minimum number of five alignments. Data were visualized in the UCSC genome browser. Accession codes: The data discussed in this publication have been deposited in NCBI's Gene Expression Omnibus and are accessible through accession number GSE52977 . How to cite this article: Yoon, J.-H. et al. PAR-CLIP analysis uncovers AUF1 impact on target RNA fate and genome integrity. Nat. Commun. 5:5248 doi: 10.1038/ncomms6248 (2014).